Marine nitrogen fixers mediate a low latitude pathway for atmospheric CO2drawdown Roughly a third (~30 ppm) of the carbon dioxide (CO 2 ) that entered the ocean during ice ages is attributed to biological mechanisms. A leading hypothesis for the biological drawdown of CO 2 is iron (Fe) fertilisation of the high latitudes, but modelling efforts attribute at most 10 ppm to this mechanism, leaving ~20 ppm unexplained. We show that an Fe-induced stimulation of dinitrogen (N 2 ) fixation can induce a low latitude drawdown of 7–16 ppm CO 2 . This mechanism involves a closer coupling between N 2 fixers and denitrifiers that alleviates widespread nitrate limitation. Consequently, phosphate utilisation and carbon export increase near upwelling zones, causing deoxygenation and deeper carbon injection. Furthermore, this low latitude mechanism reproduces the regional patterns of organic δ 15 N deposited in glacial sediments. The positive response of marine N 2 fixation to dusty ice age conditions, first proposed twenty years ago, therefore compliments high latitude changes to amplify CO 2 drawdown. As much as 30 ppm of the total glacial-interglacial difference in atmospheric CO 2 is attributed to marine biological mechanisms [1] . The most prominent biological mechanism is the fertilisation of Fe-limited high latitude regions, namely the Southern Ocean [2] and subarctic Pacific [3] , with dust-borne Fe under dusty glacial conditions [4] , [5] . Today, phytoplankton that inhabit these high latitude regions are unable to consume all available macronutrients, which allows CO 2 to escape to the atmosphere as deep waters mix into surface layers. Iron fertilisation of the high latitude glacial ocean therefore stands as a leading hypothesis to explain a more efficient biological carbon (C) pump and the associated drawdown of atmospheric CO 2 . Yet, modelling focussed on the high latitudes has sequestered less than 10 ppm of atmospheric CO 2 via Fe fertilisation [5] , [6] , [7] and indicates that additional biological mechanisms are required. There are good reasons to accommodate the lower latitudes in our search for additional mechanisms. First, the region is enormous. Surface waters between 40°S and 40°N represent over two thirds of CO 2 outgassing to the atmosphere [8] and more than half of global C export [9] , [10] . Second, unconsumed phosphate (PO 4 ) at concentrations in excess of 0.1 to 0.2 mmol m −3 exists in surface waters across the tropics, which is evidence for unrealised biological CO 2 fixation. Third, tropical oceans produce organic matter that is enriched in C because tropical phytoplankton are adapted to fix more C per unit phosphorus (P) under P scarcity [11] . Fourth, oxygen-deficient waters in the tropical Pacific, Indian and Atlantic allow organic matter to sink deeper into the ocean interior [10] , [12] , [13] . If these mechanisms are combined, the co-occurrence of more complete PO 4 utilisation and the production of C-enriched organic matter near to oxygen-deficient zones would constitute an effective pathway of CO 2 drawdown. Enabling greater PO 4 utilisation and CO 2 drawdown in the lower latitudes, however, requires simultaneously relieving Fe limitation in upwelling zones [14] , nitrate (NO 3 ) limitation in the tropics [14] , [15] and their co-limitation at the boundary of both regimes [16] . An aeolian Fe-induced stimulation of dinitrogen (N 2 ) fixation is therefore an obvious candidate to alleviate low latitude nutrient limitation. Originally proposed by Falkowski [17] , this mechanism is now supported by many independent lines of evidence. N 2 fixers are highly sensitive to the aeolian supply of Fe [18] , [19] , they represent up to half of primary production and C export in oligotrophic waters [20] , [21] , [22] , [23] , [24] , they are physiologically adapted to P scarcity [25] , [26] , produce organic matter that is enriched in C [27] , [28] , [29] , and previous modelling has demonstrated the potential of N 2 fixation to draw CO 2 into the ocean [30] . Dinitrogen fixation is also inextricably linked to suboxic zones (dissolved oxygen (O 2 ) < 10 mmol m −3 ) where denitrification strips NO 3 from the waters that upwell at the equator, creating a potential niche for N 2 fixers across the wide expanse of the lower latitudes. The strength of N 2 fixation, which strengthens PO 4 utilisation, whole community C:P ratios and C export [20] , is thus tied to the strength of denitrification, which in turn strengthens N 2 fixation. In this study, we use an ocean model to demonstrate that aeolian Fe supply to the tropical oceans under glacial conditions [31] , [32] relieves low latitude nutrient limitation [14] , [15] , [16] by stimulating N 2 fixation, which in turn drives PO 4 consumption, suboxic zone expansion, the acceleration of the nitrogen (N) cycle and a more efficient C export to the interior ocean. Furthermore, we estimate the contribution of this mechanism to CO 2 drawdown and reveal evidence of its existence within glacial-interglacial sedimentary records of N isotopes ( δ 15 N org ). A low latitude pathway Inspired by these insights, we undertook multi-millennial simulations using a global ocean biogeochemical model to explore the link between Fe fertilisation, N 2 fixation and CO 2 drawdown. The ocean biogeochemical model is part of the Commonwealth Scientific and Industrial Research Organisation (CSIRO) Mark 3L—Carbon of the Ocean, Atmosphere and Land (Mk3L-COAL) [33] . The model is designed for long-term, global oceanographic studies. It resolves multi-millennial timescales and so produces equilibrium circulation states under a given set of atmospheric conditions. It is equipped with prognostic C, PO 4 , NO 3 , 15 NO 3 , and Fe cycles [34] (see Methods), and includes a dynamic ecosystem component where phytoplankton alter their nutrient requirements, stoichiometry and remineralisation rates according to their environment [33] (Supplementary Fig. 1 ). We increased the supply of aeolian Fe to the ocean model from its modern [35] to glacial rate [5] (see Methods; Supplementary Fig. 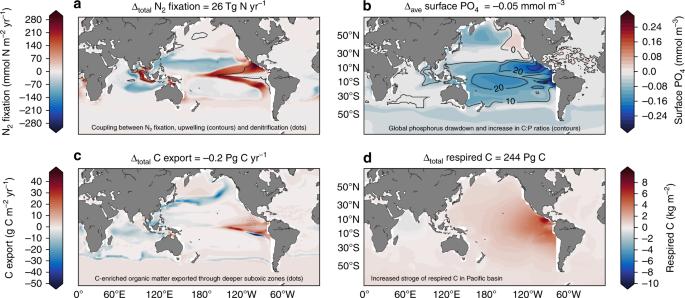Fig. 1 Biogeochemical response to an Fe-induced stimulation of N2fixers. Change inaN2fixation rate,bsurface PO4concentration,ccarbon export rate anddtotal respired carbon through the water column. The changes shown in both the coloured shading and the headings above each panel show the effect of increasing Fe deposition from the modern flux to the glacial flux5. The headings describe the integrated change (Δtotal) or the average change (Δave) of each property, calculated as the volume or area weighted sum/average of each property. Dots in (a) represent active water column denitrification. Contours in (a) define upwelling where ideal water age >25 years at 80 metres depth. Contours in (b) are the change in C:P ratios of exported organic matter. Dots (dashes) in (c) define a vertical expansion (shrinking) of suboxia >500 metres 2 ) under preindustrial physical conditions (Mk3L mild state in Table 1 ; Supplementary Note 1 ; Supplementary Figs. 3 and 4 ; Supplementary Table 1 ) with an atmospheric CO 2 held at 280 ppm, and assessed changes to elemental cycling. To isolate the response of the lower latitudes, we nudged subsurface Fe concentrations to 0.6 μmol m −3 on a yearly timescale, which ensured that Fe was near non-limiting in regions of strong mixing, like the Southern Ocean and subarctic Pacific. Table 1 Global properties of the four ocean states Full size table The glacial aeolian Fe supply increased the global rate of N 2 fixation by 26 Tg N yr −1 and caused a large-scale change in its distribution (Fig. 1a ). Dinitrogen fixers exhibited a closer coupling to regions of strong upwelling in the tropics (solid contour in Fig. 1a ) that are co-located with areas of denitrification (dots in Fig. 1a ). The greatest changes were observed in the Pacific. Dinitrogen fixation decreased in the Northwest Pacific and increased in the Eastern Tropical Pacific, which hosted low rates of N 2 fixation under modern Fe supply (Supplementary Fig. 5a ). As a result, surface PO 4 was reduced throughout the tropical Pacific by between 0.1 and 0.2 mmol m −3 (Fig. 1b ; Supplementary Fig. 5b ). Pacific PO 4 utilisation increased the C:P ratio of exported organic matter by an average of ~14 units (contours in Fig. 1b ), which elevated local C export (Fig. 1c ; Supplementary Fig. 5c ), caused a vertical expansion of suboxia (dots in Fig. 1c ), and enabled the permanent accumulation of 244 Pg of respired C in the eastern Pacific (Fig. 1d ; Supplementary Fig. 5d ). As a result, 11.6 ppm of CO 2 was permanently sequestered (see “Quantifying CO 2 drawdown” and Fig. 2 ). Fig. 1 Biogeochemical response to an Fe-induced stimulation of N 2 fixers. Change in a N 2 fixation rate, b surface PO 4 concentration, c carbon export rate and d total respired carbon through the water column. The changes shown in both the coloured shading and the headings above each panel show the effect of increasing Fe deposition from the modern flux to the glacial flux [5] . The headings describe the integrated change (Δ total ) or the average change (Δ ave ) of each property, calculated as the volume or area weighted sum/average of each property. Dots in ( a ) represent active water column denitrification. Contours in ( a ) define upwelling where ideal water age >25 years at 80 metres depth. Contours in ( b ) are the change in C:P ratios of exported organic matter. Dots (dashes) in ( c ) define a vertical expansion (shrinking) of suboxia >500 metres Full size image Fig. 2 N 2 fixation and its relationship with atmospheric CO 2 . The atmospheric reservoir of CO 2 was made responsive to oceanic uptake and release of C by the ocean (see methods). Coloured edges of markers correspond to ocean states as described in the figure legend. Star markers represent oceans with carbon cycles equilibrated to the modern Fe deposition [36] under atmospheric CO 2 of −280 ppm. The plus symbol in each ocean state represents the change due to a glacial increase in Fe supply [6] , which represents a global integrated increase of 500% over the modern supply but is regionally variable (Supplementary Fig. 2 ). Triangles represent changes in the half-saturation constant for Fe limitation of N 2 fixers, emulating changes in Fe supply to only N 2 fixers. Note the diminishing gains in CO 2 drawdown between 500 and 2500% iron deposition scenarios, consistent with Fe-saturation and PO 4 limitation. Regression lines and their slopes (gradient ± standard deviation (SD)) represent the linear relationship between N 2 fixation and atmospheric CO 2 , with a multi-ocean mean of 0.58 ± 0.03 ppm CO 2 sequestered for every additional Tg N yr −1 . Source data are provided in the source data file Full size image Dust-borne Fe fertilisation therefore involved a set of biogeochemical feedbacks, not possible by increasing the NO 3 inventory (Supplementary Note 2 ; Supplementary Fig. 6 ), that enabled CO 2 drawdown. Tropical upwelling zones are highly productive regions that drive strong subsurface O 2 depletion, which in turn stimulates denitrification and strips upwelling waters of NO 3 . Consequently, the tropical Pacific hosts low NO 3 :PO 4 ratios (Supplementary Fig. 7a ), which provides a competitive niche for N 2 fixers. Today, the low supply of aeolian Fe to the tropical Pacific [31] , [35] prevents N 2 fixers from inhabiting this niche [24] , and allows excess, unconsumed PO 4 (>0.2 mmol m −3 ) to spill 10–15° either side of the equator [36] (Supplementary Fig. 7b ). In contrast, the glacial Fe supply allowed N 2 fixers to inhabit the low NO 3 :PO 4 waters at the boundary to upwelling zones where local Fe-N co-limitation prevails today [14] , [16] . This shift in N 2 fixation initiated strong biogeochemical feedbacks that encouraged PO 4 utilisation, C export, suboxic expansion, denitrification, and a local NO 3 supply via N 2 fixation. Two consequences of this simulated feedback, the local increase in C export and a vertical expansion of suboxia, enabled the transfer of large amounts of C-rich organic matter deep within the interior of the Pacific basin (Fig. 1d ). Quantifying CO 2 drawdown We sought to quantify the sensitivity of atmospheric CO 2 drawdown to the physical conditions of the ocean, as glacial conditions were distinct from pre-industrial [37] . We produced four different ocean states that can be considered broadly representative of glacial-interglacial conditions, encompassing warm to cold, well-mixed to stratified, and thus interglacial to glacial (Table 1 ; Supplementary Fig. 8 ). Dust-borne Fe supply was varied to 50, 80, 100, 500% (glacial) and 2500% of the modern rate [35] over these four ocean states (see Methods) to fully encompass the glacial-interglacial range in conditions. Both high Fe deposition scenarios (500 and 2500%) are based on the climatology of Lambert [5] , meaning that the delivery of Fe is not uniformly greater everywhere (Supplementary Fig. 2 ). The tropical Pacific, for instance, receives roughly 2-fold more Fe than under modern conditions consistent with recent estimates [31] , [32] . In addition, we increased and decreased the Fe requirements of N 2 fixers without varying aeolian Fe deposition (See methods), which emulated variations in Fe supply but only to N 2 fixers. If similar changes occurred via both methods, then N 2 fixation could be considered the primary driver of CO 2 drawdown. The ocean states were GFDL warm , Mk3L mild (control state used previously), HadGEM cool and Mk3L cold . GFDL warm was the warmest, youngest (see δ 14 C), most deoxygenated, NO 3 -deplete and PO 4 -rich ocean, with a rapid overturning circulation dominated by the upper cell. Mk3L mild and HadGEM cool were cooler, fresher and formed greater quantities of Antarctic Bottom Water than GFDL warm . The key difference between Mk3L mild and HadGEM cool was the rate of North Atlantic Deep Water formation, which was stronger for Mk3L mild and elevated surface PO 4 , C export, O 2 consumption and denitrification rates. Mk3L cold represented full glacial conditions. It was the coldest, saltiest, and oldest ocean state, featuring strong vertical density gradients that restricted PO 4 supply and a greatly expanded lower overturning cell consistent with glacial conditions [38] . An increase in Fe supply drew between 6.7 and 16 ppm of atmospheric CO 2 into the ocean (compare star and plus symbols in Fig. 2 ). Different ocean states (colours in Fig. 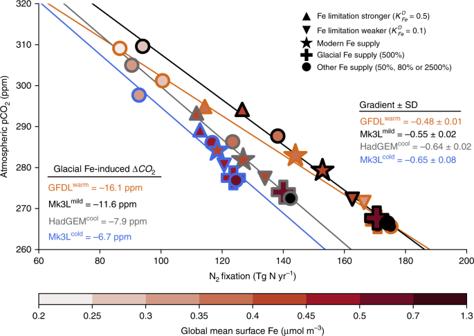Fig. 2 N2fixation and its relationship with atmospheric CO2. The atmospheric reservoir of CO2was made responsive to oceanic uptake and release of C by the ocean (see methods). Coloured edges of markers correspond to ocean states as described in the figure legend. Star markers represent oceans with carbon cycles equilibrated to the modern Fe deposition36under atmospheric CO2of −280 ppm. The plus symbol in each ocean state represents the change due to a glacial increase in Fe supply6, which represents a global integrated increase of 500% over the modern supply but is regionally variable (Supplementary Fig.2). Triangles represent changes in the half-saturation constant for Fe limitation of N2fixers, emulating changes in Fe supply to only N2fixers. Note the diminishing gains in CO2drawdown between 500 and 2500% iron deposition scenarios, consistent with Fe-saturation and PO4limitation. Regression lines and their slopes (gradient ± standard deviation (SD)) represent the linear relationship between N2fixation and atmospheric CO2, with a multi-ocean mean of 0.58 ± 0.03 ppm CO2sequestered for every additional Tg N yr−1. Source data are provided in the source data file 2 ) therefore absorbed different quantities of CO 2 . However, all states developed a positive, linear relationship between N 2 fixation and CO 2 drawdown (coloured lines in Fig. 2 ). A consistent relationship between N 2 fixation and CO 2 drawdown suggested that all states absorbed atmospheric CO 2 via the same low latitude pathway described in previously. Approximately 0.58 ± 0.03 ppm of CO 2 was absorbed by the ocean for every additional Teragram of N fixed per year (Tg N yr −1 ). The linear relationship was generated as N 2 fixation responded to variations in Fe supply (circles) and as N 2 fixation was made more or less sensitive to the modern supply of Fe (triangles). Similar responses occurred via both methods (altered Fe deposition and Fe requirements) and strongly implicated N 2 fixation as the driver of CO 2 drawdown. The sensitivity of each ocean state to changes in N 2 fixation was fundamentally linked to the strength of equatorial upwelling. The greatest sensitivity was found in GFDL warm , which featured strong upwelling, and therefore high surface PO 4 and large suboxic zones (Table 1 ). Consequently, large regions of the tropical ocean were low in NO 3 :PO 4 , which enabled large gains in N 2 fixation (88 Tg N yr −1 ) and CO 2 drawdown (43 ppm) as Fe supply increased from 50 to 2500% of its modern rate. In contrast, Mk3L cold featured the weakest rates of upwelling, lowest surface concentrations of PO 4 , the smallest suboxic zones (Table 1 ), and thus the weakest sensitivity. Phosphate availability therefore emerged as the ultimate control on biological CO 2 drawdown by setting N 2 fixation potential, while Fe supply modulated the extent to which this potential was realised. A central role for N 2 fixers The previous experiments showed that N 2 fixers responded to Fe addition leading to reduced atmospheric CO 2 . To elucidate the mechanisms through which this occurred we considered several additional experiments with the Mk3L mild ocean state subject to variations in aeolian Fe supply. First, we removed N 2 fixers and denitrification completely, thereby holding the NO 3 reservoir constant. Second, we reinstated N 2 fixers (NO 3 supply) and a marine N cycle (active denitrification), but removed their C export by setting their C:P ratio equal to zero. Third, we decreased their C:P ratio to 165:1, half its default of 331:1 [39] . Fourth, we reinstated their default C:P ratio of 331:1, but increased their PO 4 half-saturation coefficient \(\left( {K_{PO_4}^D} \right)\) to 0.1 mmol m −3 , which is the same as the general phytoplankton group and so removed their competitive advantage for PO 4 . These experiments revealed that N 2 fixers were essential for C accumulation via the low latitudes. If N 2 fixers were removed and the NO 3 reservoir remained constant, greater Fe supply did not cause respired C storage (ones in Fig. 3a ). Insensitivity to Fe supply was due to widespread NO 3 limitation of lower latitude ecosystems [15] . The simple addition of N 2 fixers without changes in Fe increased NO 3 supply to surface waters (Supplementary Fig. 9 ) and increased PO 4 utilisation between 40°S and 40°N by 7%. Dinitrogen fixers were, therefore, able to provide significant gains to the oceanic C store over millennia, which extends insights of in situ studies [20] , [21] , [22] , [23] and prior modelling [30] to the scale of the glacial cycles, as originally proposed by Falkowski [17] . Fig. 3 How N 2 fixation enables CO 2 storage in the ocean. The response of the respired C inventory to aeolian Fe deposition experiments for five different representations of N 2 fixers, with a demonstrating the relationship between respired C and Fe availability and b demonstrating the relationship between respired C and N 2 fixation. The marker numbers refer to how N 2 fixers are represented. Ones: no N 2 fixers and no active N cycle. Twos: N 2 fixers and N cycle (i.e., denitrification) reinstated but no N 2 fixer carbon export (C:P = 0:1). Threes: N 2 fixers C:P ratio increased to 165:1, half its default value. Fours: N 2 fixers PO 4 limitation enforced by increasing their half saturation coefficient \(\left( {K_{PO_4}^D} \right)\) from 10 −10 to 0.1 mmol m −3 . Fives: N 2 fixers with default parameterisation. Colour shading of the markers indicates the mean surface PO 4 concentration of the experiment. Background shading in b is a qualitative indicator of the transition from NO 3 to PO 4 limitation, where dark green to yellow indicates NO 3 limitation and light blue indicates PO 4 limitation. Source data are provided in the source data file Full size image Dinitrogen fixers were therefore essential for oceanic C storage for the simple reason that they supplied fixed N to the upper ocean. Fixed N supply was responsible for 70% of the C gains (~5–11 ppm) and responsible for the increase in PO 4 utilisation as Fe supply increased (compare ones and twos in Fig. 3a ). Included within this C storage was the increase in C:P ratios of Pacific Ocean phytoplankton as PO 4 concentrations declined (see Fig. 1b ). The final 30% (~2–5 ppm CO 2 ) of additional C gain was mostly due to export of N 2 fixer’s C-rich organic matter as the ocean became PO 4 -limited (compare ones, threes and fives in Fig. 3a ), while their efficient utilisation of PO 4 provided a small benefit to oceanic C storage (compare fours and fives in Fig. 3a ). As N 2 fixers already inhabit a niche of low NO 3 :PO 4 [20] , they are already at a competitive advantage over non-N 2 fixing phytoplankton for available PO 4 . The linear relationship between N 2 fixation and CO 2 drawdown, which was robust across different ocean states (Fig. 2 ), was therefore built on two phases. The first phase (green-yellow shading in Fig. 3b ) occurred in a NO 3 -limited ocean, where N 2 fixation increased the supply of NO 3 to surface communities and thereby allowed excess PO 4 to be consumed. The second phase (light blue shading in Fig. 3b ) occurred in a PO 4 -limited ocean. As N 2 fixers consumed proportionally more of the remaining PO 4 , their C export became more important for overall C export (compare ones, threes and fours/fives Fig. 3b ). The slope of the linear relationship presented in Fig. 2 , therefore, rested on a C:P ratio of N 2 fixer organic matter equal to 331:1 [39] . While there is significant variation around this number, under PO 4 -limiting conditions the C:P ratio tends to increase, exceeding 500:1 among Trichodesmium species [28] . Therefore, the C:P of N 2 fixers could rise as PO 4 -limiting conditions develop and steepen the linear relationship to enable greater CO 2 drawdown above that suggested here. Glacial δ 15 N records To test our proposed mechanism of low latitude CO 2 drawdown against observations, we simulated the response of the isotopic composition of organic N ( δ 15 N org ) to a glacial increase in Fe supply, and compared this response to a global compilation of glacial δ 15 N records (Supplementary Data 1 ). These experiments were completed within each ocean state presented in Table 1 , so as to isolate the effect of Fe fertilisation from the effects of physical changes. In the following, we discuss the response using the Mk3L mild ocean state, but each ocean state gave a similar response (Supplementary Fig. 10 ). An Fe-induced coupling of N 2 fixers to the upwelling zones of the eastern tropical Pacific increased δ 15 N org in the west and decreased it in the east, which broadly reproduced patterns of glacial-interglacial change throughout the Pacific basin (Fig. 4 ). The increase in the western part of the basin was due to local decreases in N 2 fixation and sedimentary denitrification, both of which lower δ 15 N. Our simulation of higher δ 15 N org in the west Pacific, therefore, supports the interpretation of a recent foraminifera-bound record in the South China Sea [40] (star marker). However, the simulated decrease in the δ 15 N of the eastern Pacific was not caused by a decrease in water column denitrification as suggested by numerous studies since the seminal paper of Ganeshram et al. [41] . Instead, our simulated decrease in eastern δ 15 N org was caused by increases in both sedimentary denitrification and N 2 fixation (Fig. 1a ). Fig. 4 Seeking evidence from sedimentary δ 15 N org records. Shading depicts the simulated change in δ 15 N of organic matter as a result of increasing aeolian Fe supply from the modern to a glacial rate. Solid and dashed contour lines mark simulated differences of 1 and −1. Circles mark locations of sediment cores where bulk organic matter was analysed for δ 15 N, while stars mark locations where either foraminifera- or diatom-bound δ 15 N was measured. The colour of the markers is an estimate of the glacial (Last Glacial Maximum: 20,000–26,000 BCE) minus interglacial (Late Holocene: 0–5000 BCE) difference in δ 15 N org , with red colours representing higher values and blues representing lower values in the glacial ocean. Sedimentary record data are provided in Supplementary Data 1 Full size image However, poor agreement was found in other regions, namely in the tropical western Atlantic and Southern Ocean where an increase in δ 15 N org was not simulated. In the west Atlantic, Straub et al. [42] presented a compelling relationship between δ 15 N and orbital precession, leading the authors to surmise a dependence on the upwelling of PO 4 via changes in the circulation. In the Southern Ocean, a glacial increase in δ 15 N in Subantarctic [2] and Antarctic zones [43] , [44] is explained by a weaker physical delivery of NO 3 to the mixed layer combined with Fe fertilisation. We therefore expected and found no response in both regions in these experiments (Supplementary Fig. 10 ) because the only change was an increase in dust-borne Fe and the Southern Ocean was made insensitive to increases in Fe supply. Our study confirms that N 2 fixation is a key component of the global C cycle. We extend a theoretical proposal made over 20 years ago [17] to a quantifiable mechanism of CO 2 drawdown. The main biogeochemical feedbacks are illustrated in Fig. 5 , where a coupling of N 2 fixers to upwelling zones is the catalyst that drives CO 2 drawdown. Fig. 5 Scenarios of Fe supply to the tropical Pacific. In the low iron scenario, analogous to the modern climate, N 2 fixation (yellow zone and dots) is concentrated in the Northwest and Southwest subtropical Pacific where aeolian dust deposition is greatest. Non-limiting PO 4 concentrations (green zone and dots) exist within the tropics and spread laterally from the area of upwelling near the Americas and at the equator (blue zone). In the high Fe scenario, analogous to the glacial climate, N 2 fixation couples to the upwelling zones in the east Pacific, enabling strong utilisation of PO 4 , the vertical expansion of suboxic zones (grey bubbles) and a deeper injection of carbon-enriched organic matter (downward squiggly arrows) Full size image The importance of N 2 fixation for CO 2 drawdown is relevant when assessing prior modelling work. Simulations of the glacial climate have struggled to explain the full drawdown of roughly 90 ppm [45] , unless they make manual, and therefore non-mechanistic, changes to biological functioning [38] , [46] . Furthermore, model studies that explore Fe fertilisation without considering variable stoichiometry and remineralisation rates [6] , [7] have struggled to sequester more than 10 ppm of CO 2 . The permanent sequestration of 7–16 ppm solely via the low latitudes, therefore, represents a new and complementary pathway to explain the glacial CO 2 drawdown. Thinking conservatively given the stratified and therefore PO 4 -limited conditions of a glacial ocean [37] , [42] , we propose that one third, or 10 ppm, of the 30 ppm attributed to Fe fertilisation [1] can be explained by a closer coupling of N 2 fixation to tropical upwelling zones. It is important to recognise, however, that our simulations rendered eutrophic regions insensitive to Fe fertilisation. Consequently, we neglect the response of Fe-limited regions like the Southern Ocean that not only have demonstrated potential for CO 2 drawdown [5] , [6] , [7] , [38] , [45] , but also influence low latitude biogeochemistry through mode and intermediate waters [47] . This work should therefore not be interpreted as a globally integrated response to Fe fertilisation. Instead, it isolates the response of the lower latitudes and offers important lessons. First, that the debated [32] , [48] , [49] CO 2 drawdown via the tropics is possible. Second, that this drawdown can accompany and thus complement high latitude mechanisms of CO 2 drawdown. Third, that this drawdown requires simultaneous relief from both Fe and NO 3 limitation [14] , [15] , [16] , which is plausibly achieved by stimulating N 2 fixers with dust-borne Fe. Our confidence in this N 2 fixer-mediated mechanism is bolstered by our simulation of the glacial-interglacial changes in δ 15 N org within the Pacific basin. However, both the drawdown of CO 2 and the reproduction of the δ 15 N org patterns in our study hinge on an acceleration of N cycling in the Eastern Tropical Pacific. By acceleration of N cycling, we mean an acceleration of the rates of N 2 fixation and denitrification. Such an acceleration conflicts with a long-assumed deceleration of N cycling. Since Ganeshram et al. [41] , glacial records of low δ 15 N org are interpreted to reflect a massive deceleration of water column denitrification, which must have exceeded a deceleration of sedimentary denitrification caused by a loss of shelf area [50] . Instead, our simulations produced an increase in sedimentary denitrification under Fe fertilisation. While both possibilities can explain the trends in Pacific δ 15 N org because they both involve more sedimentary over water column denitrification, they diverge in the inferred intensity of N cycling. New evidence questions a glacial deceleration of the N cycle in the Eastern Tropical Pacific. Recent work has revealed a vertical expansion of Pacific suboxic zones [32] , [51] , a feature reproduced by our Fe fertilisation simulations. While it is not well known whether sedimentary or water column denitrification is more sensitive to increases in suboxia, it seems unlikely that both would decrease as suboxic zones expanded. In fact, it seems more likely that sedimentary denitrification was stimulated as waters overlying the sediment became deoxygenated [52] and as more organic carbon was buried within sediments [53] , while water column denitrification, which is centred within the thermocline [54] , was reduced in line with reduced rates of particle export [55] . If suboxic zones did expand vertically [32] , [51] , [52] and local N cycling accelerated, then the coupling of N 2 fixers to eastern upwelling zones and subsequent CO 2 drawdown is legitimate. The legitimacy of our proposal then requires explaining another apparent inconsistency in glacial records: how could less particle export [55] in the tropical Pacific coincide with more C export? Our results suggest that an answer may be found in the combination of variable stoichiometry and deoxygenation. Strong PO 4 utilisation and aeolian Fe supply enriches the C content of exported organic matter [11] , [56] , while deoxygenation enables a strong transfer of particles to depth [10] , [12] , [13] . If both features were present during glacial periods, then lower rates of particle export [55] do not preclude more C export, and therefore CO 2 drawdown. Today, there are compelling signs that N 2 fixation has strengthened within the Pacific since the industrial revolution [57] , [58] and that suboxic zones are expanding [59] , [60] . Our experiments suggest that these changes are symptomatic of a stronger biological C pump, but even so, we propose that gains in N 2 fixation remain unrealised. Evidence that N 2 fixation is operating well below full capacity can be found in the excess PO 4 that spreads 10–15° outwards from tropical upwelling zones [36] (Supplementary Fig. 7b ) and the spatial decoupling of N 2 fixation from denitrification [24] . Realising the full potential of N 2 fixation appears primarily dependent on the delivery of aeolian Fe to the surface ocean. Like the high latitudes [2] , [3] , we find that the strength of the lower latitude biological C pump demonstrates a strong link to the Fe cycle. However, how the oceanic Fe cycle will change in the future is uncertain [61] , and undermines our ability to predict the ocean’s role in atmospheric CO 2 drawdown in the coming centuries. Model Model simulations were performed using the ocean component of the Commonwealth Scientific and Industrial Research Organisation (CSIRO) Mark 3L—Carbon of the Ocean, Atmosphere and Land (Mk3L-COAL) Earth system model. The ocean component is comprised of an ocean general circulation model (OGCM) described in Phipps et al. [62] and an ocean biogeochemical model (OBGCM) described in Buchanan et al. [33] and Buchanan et al. [34] . A more specific description of the N cycle and Fe cycle are presented in the supplement. The ocean model has a horizontal resolution of 2.8° in longitude by 1.6° in latitude, with 21 vertical levels. It is a coarse resolution, z -coordinate OGCM, allowing millennial timescales to be resolved. The OBGCM is equipped with 13 prognostic tracers that can be grouped into carbon chemistry fields, oxygen fields, nutrient fields and age tracers. Carbon chemistry and air-sea gas exchange is parameterised according to the latest ocean model requirements [63] . Nitrogen isotope routines are described in Buchanan et al. [34] . The cycling of organic matter considers three forms of phytoplankton. These are a general phytoplankton group ( G ), N 2 fixers (otherwise known as diazotrophs; D ) and calcifiers. The general phytoplankton group is controlled by dynamic equations for organic matter production, remineralisation and stoichiometry according to the study of Buchanan et al. [33] . These equations allow the general phytoplankton group to represent variations in the biogeochemical properties of the marine ecosystem, which has positive effects on the simulation of global ocean biogeochemistry, particularly the N cycle. Meanwhile, N 2 fixers and calcifiers follow more static equations. N 2 fixers have fixed nutrient limitation functions and stoichiometry based on laboratory studies, but are also remineralised according to community composition. Remineralisation of both forms of organic matter is also conserved and passed to deeper grid boxes if oxygen is not sufficient. The calcifying group, which only interacts with DIC and ALK species, produces particulate inorganic carbon at 8% of the rate at which the general phytoplankton group produces organic carbon. Its remineralisation rate is also fixed according to an e -folding depth-dependent decay, which transfers a large fraction of particulate inorganic carbon to the deep ocean. Nitrogen cycle Nitrate is introduced to the ocean through atmospheric deposition and N 2 fixation. Atmospheric deposition adds 11.3 Tg N to the surface ocean each year using a prescribed monthly climatology [64] . The addition of NO 3 by N 2 fixation is calculated by considering marine N 2 fixers as a unique group of phytoplankton. N 2 fixers consume PO 4 and Fe at the surface ocean, and release PO 4 , Fe and NO 3 at depth during remineralisation. The stoichiometry of N 2 fixers is static, with a C:N:P:Fe ratio of 331:50:1:0.00064 according to physiological studies [39] , [65] , [66] . With this stoichiometry, we apply O rem :P and N rem :P requirements of 431 and 294.8, respectively, using the equations of Paulmier et al. [67] . The export of phosphorus by N 2 fixers \((P_{exp}^D)\) is calculated using a maximum growth rate μ D ( T ) that is temperature dependent [68] , limitation terms dependent on the availability of PO 4 , NO 3 and Fe, and minimum thresholds to account for cold water N 2 fixation [69] . These terms are applied against an export:production ratio \((S_{E:P}^D)\) in units of mmol P m −3 day −1 . \(P_{exp}^D\) is calculated via: 
    P_exp^D = S_E:P^D ·μ ^D(T) ·max(0.01,min(PO_4_lim^D,NO_3_lim^D,Fe_lim^D)) · (1 - ico)
 (1) where, 
    μ ^D(T) = max(0.01, - 0.0042T^2 + 0.2253T - 2.7819)
 
    PO_4_lim^D = PO_4/PO_4 + K_PO_4^D
 
    NO_3_lim^D = e^ - NO_3
 
    Fe_lim^D = max(0.0, 1pttanh(2Fe - K_Fe^D))
 The Fe half saturation coefficient ( \(K_{Fe}^D\) ) was kept at 0.3 μmol m −3 , 3× that of other phytoplankton, unless otherwise clearly defined as another value in our discussion of the results below. The PO 4 half saturation coefficient ( \(K_{PO_4}^D\) ) was 10 −10 unless otherwise clearly defined as another value to emulate N 2 fixers efficient utilisation of P [25] , [26] . Light was also not considered as a limiting factor. A dependency on light was omitted because of the strong correlation between incident radiation and sea surface temperature [70] and its negligible effect on N 2 fixation in the Atlantic Ocean [71] . Finally, the fractional area coverage of sea ice ( ico ) is included to ensure that no cool-water N 2 fixation [69] occurs under ice. The remineralisation of N 2 fixer export occurs at the same rate as other labile organic matter produced by the general phytoplankton group. Two processes remove NO 3 from the ocean model: water column and sedimentary denitrification. Water column denitrification occurs when O 2 concentrations are less than a particular threshold \((R_{lim}^{O_2})\) , which is set at 7.5 mmol O 2 m −3 . We calculate the fraction of organic matter ( P org ) that is remineralised by water column denitrification via: 
    f_den = ( 1 - e^ - 0.5 · R_lim^O_2 + e^O_2 - 0.5 · R_lim^O_2)^ - 1
 (2) and then apply the appropriate stoichiometric requirements of NO 3 to this fraction of P org : 
    Δ NO_3(WC_den) = f_den· P_org·N_rem:P
 (3) Following this, the strength of water column denitrification is reduced if the ambient concentration of NO 3 is deemed to be limiting. Water column denitrification depletes NO 3 towards concentrations between 15 and 40 mmol m −3 in modern suboxic zones [36] . Without this additional constraint, here defined as r den , NO 3 concentrations quickly go to zero in simulated suboxic zones. We calculate r den by prescribing a lower limit at which NO 3 can no longer be consumed \((R_{lim}^{NO_3})\) , which was set to 30 mmol NO 3 m −3 : 
    r_WC_den = 0.5 + 0.5 ·tanh(0.25 ·NO_3 - 0.25 · R_lim^NO_3 - 2.5)
 (4) 
    if   r_WC_den <  3pt f_den,  then   f_den = r_WC_den
 (5) Sedimentary denitrification was calculated using the paramaterisation of Bohlen et al. [72] , where the removal of NO 3 is dependent on the rain rate of organic carbon to the sediments ( C org ) and the ambient concentrations of O 2 and NO 3 . ΔNO_3(S_den) = ( α + β· 0.98^(O_2 - NO_3)) · C_org
 (6) The α term was 0.08, while the β term was halved compared the original value of Bohlen et al. [72] to β = 0.1 in an attempt to increase the deep NO 3 inventory. The availability of NO 3 for sedimentary denitrification was accounted for according to the equation: 
    r_S_den = 0.5 + 0.5 ·tanh(10 ·NO_3 - 5)
 (7) Thus, sedimentary denitrification was relaxed towards zero as NO 3 concentrations became low. If NO 3 was limiting, the remaining organic matter was remineralised using O 2 , so long as the environment was sufficiently oxygenated. The availability of oxygen in the sediments was estimated to be two-thirds of the overlying bottom water concentration, based on observations of transport across the diffusive boundary layer by Gundersen and Jorgensen [73] . Furthermore, an additional limitation was set for sediments underlying hypoxic waters (O 2 < 40 mmol m −3 ), where aerobic remineralisation was diminished towards zero according to the hyperbolic tangent function: 
    r_S_rem = 0.5 + 0.5 ·tanh(0.2 ·O_2 - 5)
 (8) If both NO 3 and O 2 were limiting, the remaining organic matter was assumed to be remineralised via sulfate reduction. Subgrid-scale bathymetry A large amount of sedimentary remineralisation was not included using these parameterisations because the coarse resolution OGCM enables it to resolve only the largest continental shelves. Many small areas of raised bathymetry in pelagic environments were also unresolved. To address this insufficiency, we coupled a sub-grid scale bathymetry to the course resolution OGCM following the methodology of Somes et al. [74] and using the ETOPO5 \(\frac{1}{{12}}^{th}\) of a degree dataset. For each latitude by longitude grid point, we calculated the fraction of area that would be represented by shallower levels in the OGCM if this finer resolution bathymetry were used. At each depth level above the OGCM’s deepest level, the fractional area represented by sediments on the sub-grid scale bathymetry was used to remineralise all forms of organic matter via the sedimentary processes defined above. Iron cycle Our simulated Fe cycle involves a prescribed external source via the aeolian deposition of dust [35] , and an internal control in water masses in contact with the ocean floor. The internal control relaxes Fe concentrations to a set concentration given in the control file, which is set to 0.6 μmol m −3 over a period of 1 year. The iron cycle, therefore, considers an atmospheric source, internal cycling via organic matter, and deep ocean sources and sinks via the sediments. 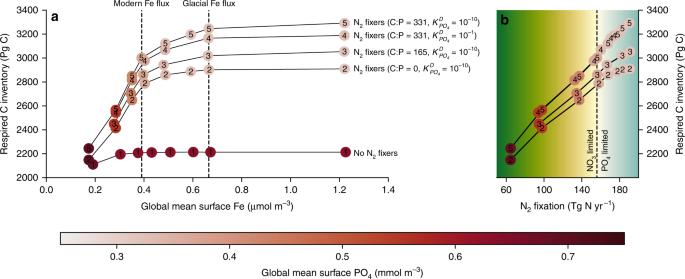Fig. 3 How N2fixation enables CO2storage in the ocean. The response of the respired C inventory to aeolian Fe deposition experiments for five different representations of N2fixers, withademonstrating the relationship between respired C and Fe availability andbdemonstrating the relationship between respired C and N2fixation. The marker numbers refer to how N2fixers are represented. Ones: no N2fixers and no active N cycle. Twos: N2fixers and N cycle (i.e., denitrification) reinstated but no N2fixer carbon export (C:P = 0:1). Threes: N2fixers C:P ratio increased to 165:1, half its default value. Fours: N2fixers PO4limitation enforced by increasing their half saturation coefficient\(\left( {K_{PO_4}^D} \right)\)from 10−10to 0.1 mmol m−3. Fives: N2fixers with default parameterisation. Colour shading of the markers indicates the mean surface PO4concentration of the experiment. Background shading inbis a qualitative indicator of the transition from NO3to PO4limitation, where dark green to yellow indicates NO3limitation and light blue indicates PO4limitation. Source data are provided in the source data file Simulations All experiments were simulated for 10,000 years to achieve steady-state solutions of major biogeochemical tracers. Unless clearly defined otherwise, all experiments were run under preindustrial conditions, Mk3L mild , driven by monthly climatologies of surface conditions over an annual cycle. Surface climatologies required to force the OGCM and OBGCM under Mk3L mild conditions were generated by a 10,000 year pre-industrial (PI) control run of the flux corrected CSIRO Mk3L v1.2 climate system model in fully coupled mode [62] . We forced the OGCM with three sets of additional boundary conditions to generate cold, cool and warm ocean states in addition to Mk3L mild . The glacial ocean state (Mk3L cold ) was generated by forcing the CSIRO Mk3L climate system model with glacial conditions as simulated in Buchanan et al. [38] . Warm and mild conditions of GFDL warm and HadGEM cool , respectively, were provided by the pre-industrial control runs of the GFDL-ESM2G and HadGEM2-CC climate system models from the Climate Model Inter-comparison Project phase 5 (CMIP5) multi-model ensemble [75] . More thorough physical analyses of these ocean states are contained in Buchanan et al. 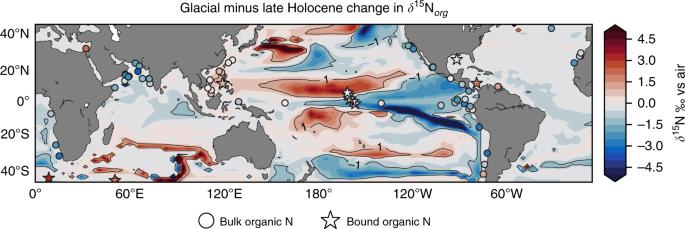Fig. 4 Seeking evidence from sedimentaryδ15Norgrecords. Shading depicts the simulated change inδ15N of organic matter as a result of increasing aeolian Fe supply from the modern to a glacial rate. Solid and dashed contour lines mark simulated differences of 1 and −1. Circles mark locations of sediment cores where bulk organic matter was analysed forδ15N, while stars mark locations where either foraminifera- or diatom-boundδ15N was measured. The colour of the markers is an estimate of the glacial (Last Glacial Maximum: 20,000–26,000 BCE) minus interglacial (Late Holocene: 0–5000 BCE) difference inδ15Norg, with red colours representing higher values and blues representing lower values in the glacial ocean. Sedimentary record data are provided in Supplementary Data1 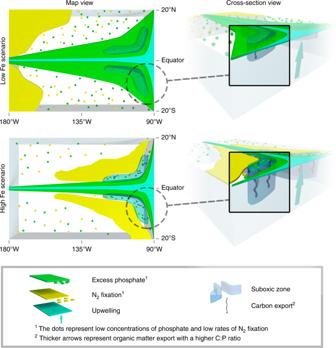Fig. 5 Scenarios of Fe supply to the tropical Pacific. In the low iron scenario, analogous to the modern climate, N2fixation (yellow zone and dots) is concentrated in the Northwest and Southwest subtropical Pacific where aeolian dust deposition is greatest. Non-limiting PO4concentrations (green zone and dots) exist within the tropics and spread laterally from the area of upwelling near the Americas and at the equator (blue zone). In the high Fe scenario, analogous to the glacial climate, N2fixation couples to the upwelling zones in the east Pacific, enabling strong utilisation of PO4, the vertical expansion of suboxic zones (grey bubbles) and a deeper injection of carbon-enriched organic matter (downward squiggly arrows) [38] and Buchanan et al. [33] . Iron deposition experiments that varied Fe supply to the surface ocean involved altering the field of Mahowald et al. [35] with constant factors to achieve 25, 50, 75, 80, 90, 100, 125, 150, 200, 300, and 400% of the modern flux. Higher fluxes representative of the glacial field were undertaken using the dust deposition fields of Lambert et al. [5] assuming 3.5% Fe content and 0.4 and 2% solubility, respectively, to achieve 500 and 2500% of the modern Fe supply rate (Supplementary Fig. S2 ). The glacial dust deposition rate referred to in the main text is the 500% version of the Lambert et al. [5] field (Supplementary Fig. 2 ). These rates of Fe deposition were applied to the Mk3L mild state and discussed in “A central role for N 2 fixers”, while a subset of these Fe deposition experiments, as well as variations in the Fe half-saturation constant for N 2 fixers (see Supplementary description of the N cycle), were undertaken in with multiple physical states discussed in “Quantifying CO 2 drawdown”. For those experiments with a freely evolving atmospheric CO 2 concentration (within section “Quantifying CO 2 drawdown”), we initialised each with the near-equilibrium solution produced by holding atmospheric p CO 2 at 280 ppm and with the modern Fe deposition (stars in Fig. 2 ), such that experiments with modern Fe deposition maintained atmospheric p CO 2 near to 280 ppm. Altering Fe deposition then caused changes in air-sea CO 2 exchange that altered the atmospheric and oceanic C reservoirs. The atmospheric C reservoir was calculated assuming a constant atmospheric weight of 5.1 × 10 21 g and a mean molecular weight of air of 28.97 g mol −1 . All experiments involved a relaxation of deep ocean Fe to values of 0.6 μmol m −3 over a period of 365 days. Areas of connection between the deep and surface ocean, such as the high latitudes and deep upwelling zones, were therefore either non-Fe limited or almost non-Fe limited. This parameterisation rendered the high latitudes insensitive to greater Fe supply, while stratified lower latitudes were sensitive to Fe supply but NO 3 -limited. δ 15 N org records Glacial minus interglacial values of δ 15 N org records were calculated by averaging values during the Last Glacial Maximum, defined as between 20 and 26 kya, and the Late Holocene, defined as between 0–5 kya. The early Holocene was ignored due to transient changes in the δ 15 N records since the deglaciation. The global compilation of δ 15 N org was composed of bulk sediment and diatom- and foraminifera-bound measurements, and is available in the supplementary material. A slight correction to simulated δ 15 N org was applied to correct for diagenetic effects that increase with depth in the water column. The addition of 0.9 per 1000 metres to the raw, simulated δ 15 N org values was applied and substantially improves comparisons between simulated and coretop values [34] .